Chemical vapour deposition growth of large single crystals of monolayer and bilayer graphene The growth of large-domain single crystalline graphene with the controllable number of layers is of central importance for large-scale integration of graphene devices. Here we report a new pathway to greatly reduce the graphene nucleation density from ~10 6 to 4 nuclei cm −2 , enabling the growth of giant single crystals of monolayer graphene with a lateral size up to 5 mm and Bernal-stacked bilayer graphene with the lateral size up to 300 μm, both the largest reported to date. The formation of the giant graphene single crystals eliminates the grain boundary scattering to ensure excellent device-to-device uniformity and remarkable electronic properties with the expected quantum Hall effect and the highest carrier mobility up to 16,000 cm 2 V −1 s −1 . The availability of the ultra large graphene single crystals can allow for high-yield fabrication of integrated graphene devices, paving a pathway to scalable electronic and photonic devices based on graphene materials. Graphene has emerged as an exciting, atomically thin two-dimensional material for fundamental studies and potential applications in future electronics [1] , [2] , [3] , [4] , [5] , [6] , [7] , [8] . The pristine graphene can be obtained through a mechanical exfoliation approach to break the weak van der Waals forces between the adjacent layers of graphite [9] . This approach can produce the best-quality graphene, but often with sizes limited in a few to a few tens of micrometres [10] . On the other hand, large-area mono- or few-layer graphene can now be readily obtained through a carbon segregation process on carbon-containing substrates (for example, SiC) or chemical vapour deposition (CVD) process on metal foils (for example, Ni or Cu) [11] , [12] , [13] . In particular, the CVD approach can be used to produce continuous mono- or few-layer graphene with the sizes measured by square metres [14] , but typically with a polycrystalline structure and a high density of domain/grain boundaries, leading to highly variable electronic properties [8] . Even though it has been reported that mobility of the CVD graphene within single domain can be comparable to the best-reported exfoliated sample, the overall transport characteristics of wafer-scale CVD graphene is still largely limited by the crystal defects at domain boundaries [15] , [16] . Therefore, to produce large graphene single crystals represents a central challenge for the large-scale integration of functional electronic and optoelectronic devices from graphene. The typical size of CVD graphene domains is on the order of 10 μm, which is dictated by the relatively large number of graphene nuclei (~10 6 cm −2 ) at the initial nucleation stage [17] , [18] . Therefore, the key challenge to achieve large-domain single crystalline graphene in a CVD process is to reduce the nucleation density. A common strategy to reduce the nucleation density is to minimize the impurity or defect density on copper surface through some relatively arduous pretreatments (for example, surface polishing and high-temperature lengthy annealing under high flow of H 2 ) of the copper substrate. For example, a long-duration (3 h) annealing of copper foils at the atmospheric pressure can be used to reduce the nucleation density to achieve 1.3-mm-sized graphene domains [19] . An electrochemically polished copper foil followed by a 7-h pre-annealing step in high flow of hydrogen gas at high temperature and high pressure can be used to prepare the copper foil for the growth of single crystalline graphene domains with sizes reaching up to 2.3 mm (ref. 20 ). Here we report a new pathway to reduce the graphene nucleation density by maintaining a catalytic inactive Cu 2 O layer during the initial nucleation stage. Our systematic studies define an integrated strategy, using pregrowth ramping/annealing in non-reducing environment, low reactor pressure and high hydrogen/methane molar ratio, to significantly suppress the graphene nucleation density by more than five orders of magnitude and reach an ultra-low density of 4 nuclei cm −2 . Using the optimized growth conditions, we demonstrate the growth of single crystalline monolayer graphene domain with a lateral size up to 5 mm and Bernal-stacked (AB-stacked) bilayer graphene domain with the lateral size up to 300 μm, both are the largest single crystalline domain sizes achieved to date, respectively. Electrical transport studies, including sheet resistance measurements, transistor studies and quantum Hall measurements, demonstrate that our graphene single crystals exhibit excellent electronic properties with the carrier mobility up to 16,000 cm 2 V −1 s −1 , and expected quantum Hall effect for both the monolayer and AB-stacked bilayer graphene. Furthermore, mobility mapping studies demonstrate that the formation of large graphene monodomain can enable excellent device-to-device uniformity that is not possible with polydomain samples. The availability of the giant graphene single crystals can allow for the implementation of high-performance graphene-based devices with excellent uniformity and reproducibility. Growth of large single crystals of monolayer graphene Scanning electron microscopy (SEM) images ( Fig. 1a ), photograph ( Fig. 1c ) and optical microscopy images ( Fig. 1d–f ) show the ultra-large single crystals of monolayer graphene obtained with a growth duration of 6, 24 and 48 h, respectively. The detailed growth procedures are described in the Methods section. The lateral size of the largest monodomain graphene can reach up to 5 mm ( Fig. 1c ). All the graphene domains shown in the SEM and optical microscopy images have a hexagonal shape with straight edges and clear uniform colour contrast. Small domains of bilayer or multilayer graphene are also occasionally seen at the centre of individual graphene domain ( Fig. 1e ). 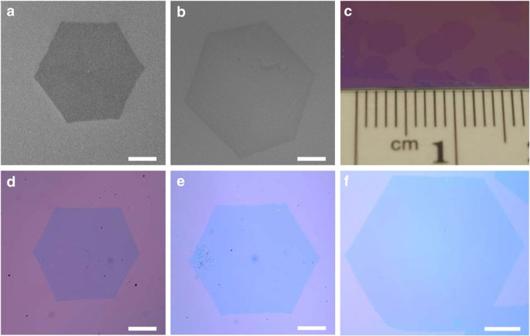Figure 1: Giant graphene single crystals obtained at variable growth durations. (a) SEM image and (d) optical microscopy image of a graphene domain obtained with 6 h of growth. (b) SEM image and (e) optical microscopy image of a graphene domain obtained with 24 h of growth. (c) Photograph and (f) optical microscopy image of graphene domains obtained with 48 h of growth. Scale bars, 0.2 mm inaandd, 0.4 mm inbande, and 1 mm inf. Figure 1: Giant graphene single crystals obtained at variable growth durations. ( a ) SEM image and ( d ) optical microscopy image of a graphene domain obtained with 6 h of growth. ( b ) SEM image and ( e ) optical microscopy image of a graphene domain obtained with 24 h of growth. ( c ) Photograph and ( f ) optical microscopy image of graphene domains obtained with 48 h of growth. Scale bars, 0.2 mm in a and d , 0.4 mm in b and e , and 1 mm in f . Full size image We have conducted a systematic investigation on the growth parameters to achieve the 5-mm-sized single crystalline graphene domains. First, we demonstrate the average domain density of the as-grown graphene can be reduced from ~5 × 10 5 to ~1 × 10 5 nuclei cm −2 when the reactor pressure is decreased from atmospheric pressure to 1 mbar ( Supplementary Figs S1 and S2 ), which is consistent with previous studies [21] , [22] . Second, we found that a ramping up (~20 min) and a short-duration annealing (~5 min) of the copper foils in non-reducing environment (for example, pure argon gas) can significantly suppress the nucleation density of graphene domains. The oxidation of the copper surface is believed to have an essential role here. A cuprous oxide (Cu 2 O) layer usually exists on the copper foils exposed to the ambient environment ( Supplementary Fig. S3 ). Our studies show that the domain density can be reduced by nearly two orders of magnitude when the copper foil is ramped up/annealed in the pure argon gas (~10 3 nuclei cm −2 ) compared with that ramped up/annealed in the argon/hydrogen mixture (~10 5 nuclei cm −2 ; Supplementary Figs S4 and S5 ). This effect is repeatedly observed in over 40 similar growth runs. The reduction of the graphene nucleation density here could be attributed to higher nucleation barrier on the copper oxide compared with the fresh copper surface. To further confirm our hypothesis, we have conducted a systematic investigation of the nucleation density dependence on the pregrowth annealing in Ar/H 2 mixture. In this study, we first annealed the copper foil in an Ar/H 2 mixture at variable temperatures for different durations before it was ramped up (in Ar) to the growth temperature for graphene growth ( Supplementary Fig. S4 ). The nucleation density was investigated after a 15-min growth process ( Supplementary Figs S5 and S6 ). The hypothesis is that the native oxide on Cu foil can be increasingly reduced back to Cu with increasing annealing temperature or duration in Ar/H 2 . The reduced Cu is catalytically more active to allow much faster and higher density nucleation of graphene domain. Indeed, our studies clearly demonstrate that graphene domain density increases with the Ar/H 2 annealing temperature or duration ( Supplementary Figs S5 and S6 ), which is in stark contrast to long-duration hydrogen annealing under high pressure (to reduce defect density and therefore nucleation density, as reported in ref. 20 ). These studies clearly demonstrate that the surface oxide plays a critical role in suppressing the nucleation of graphene on Cu surface. Once a small amount of hydrogen is introduced into the reactor, the hydrogen gas can quickly reduce the copper oxides into pure copper, due to a relatively low activation energy [23] , [24] . As the graphene tends to nucleate on reduced Cu surfaces instead of the catalytic inactive Cu 2 O surface, the nucleation density of the graphene can be greatly suppressed by maintaining the oxide layer during the initial nucleation stage. Indeed, our studies demonstrate an approximately two orders of magnitude decrease in the graphene nucleation density by avoiding the reduction of Cu 2 O surface before growth. The nucleation of graphene on copper foil can be further controlled by the molar ratios between the methane and hydrogen gases. Our studies show that a higher hydrogen/methane molar ratio leads to both a reduced nucleation density and a lower growth rate. For a constant growth duration (for example, 2 h), the graphene nucleation density can be decreased from ~10 3 nuclei cm −2 to as low as 4 nuclei cm −2 by increasing the molar ratio of H 2 /CH 4 from ~1,466 to ~6,600 ( Supplementary Fig. S7 ). The growth of graphene is believed to be a competing process between the pyrolysis of hydrocarbons and the etching effect by hydrogen. The growth of the graphene domains is sustained by continuously feeding the active carbon species from catalytic pyrolysis of hydrocarbons on copper surface. At same time, the hydrogen gas can also decompose on the copper surface to form active atomic hydrogen, which can act as an etching agent to graphene [25] , [26] , [27] . The higher H 2 /CH 4 molar ratio suppresses the graphene nucleation due to the etching effect. Together, integrating these different strategies we have greatly reduced the nucleation density down to 4 nuclei cm −2 , enabling us to achieve giant graphene single crystals with the largest area exceeding 16 mm 2 . Structural characterization We have conducted transmission electron microscopy (TEM) and electron diffraction studies to confirm the single crystalline nature of the large hexagonal graphene domains. To this end, the as-grown graphene films were transferred onto an amorphous carbon-covered TEM grid (with 100 × 100-μm-sized square holes). An SEM image of the graphene on TEM grid shows that a 1.5-mm graphene domain retains its structural integrity with the hexagonal shape well preserved ( Fig. 2a ). 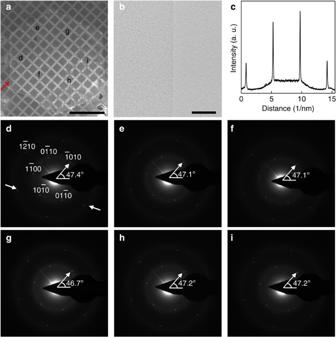Figure 2: Structural characterization. (a) SEM image of a 1.5-mm-sized monolayer graphene domain on a TEM grid with an array of 100 × 100 μm windows. Scale bar, 0.5 mm. (b) A bright-field TEM image of the graphene on the TEM grid taken from the approximate location pointed by a red arrow in panela. Scale bar, 200 nm. (c) Profile plots of the diffraction peak intensities along the white arrows ind. (d–i) SAED patterns taken from different holes of the TEM grid, labelled according to the locations indicated in panela. The white colour angle lines highlight the graphene lattice orientation (the angle between the [010] direction and thexaxis) at different locations. The relative angle of graphene lattice extracted from the SAED patterns shows less than 1.2° rotation throughout the entire domain. Figure 2b shows a bright-field TEM image of the graphene membrane at the edge region (highlighted by a red arrow in Fig. 2a ). The graphene membrane is clean, uniform, and the edge is straight. Figure 2: Structural characterization. ( a ) SEM image of a 1.5-mm-sized monolayer graphene domain on a TEM grid with an array of 100 × 100 μm windows. Scale bar, 0.5 mm. ( b ) A bright-field TEM image of the graphene on the TEM grid taken from the approximate location pointed by a red arrow in panel a . Scale bar, 200 nm. ( c ) Profile plots of the diffraction peak intensities along the white arrows in d . ( d – i ) SAED patterns taken from different holes of the TEM grid, labelled according to the locations indicated in panel a . The white colour angle lines highlight the graphene lattice orientation (the angle between the [ 010] direction and the x axis) at different locations. The relative angle of graphene lattice extracted from the SAED patterns shows less than 1.2° rotation throughout the entire domain. Full size image To confirm the crystallinity of the large graphene domain, we have conducted selective area electron diffraction (SAED) on the graphene domain at 18 selected openings ( Supplementary Fig. S8 ). Figure 2d–j shows six representative SAED patterns, with the zone axis of [0001], taken at the holes that are labelled correspondingly in Fig. 2a . The line profiles of the diffraction patterns show a diffraction intensity ratio of the outer {1120} peak over the inner {1100} peak close to 0.5, demonstrating the monolayer nature of the graphene domain ( Fig. 2c ). We extensively analysed all the diffraction patterns obtained from 18 individual window openings and found no signs of noticeable graphene boundaries or any intrinsic large-scale defects or disorder. The relative angle of graphene lattice extracted from the SAED patterns shows less than 1.2° rotation of the graphene lattice direction throughout the entire domain ( Supplementary Fig. S8 ). These results unambiguously confirm that the graphene domain is a single crystalline monolayer across its entire area. Electronic properties To evaluate the electronic quality of the giant graphene single crystals, a monodomain graphene was transferred onto 300 nm SiO 2 /Si substrate to fabricate Hall bar devices without any domain boundaries for detailed electronic property characterizations. 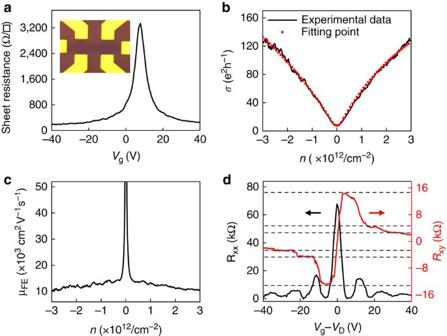Figure 3: Electronic properties. (a) Resistivity of graphene depending on the back-gate voltage at room temperature. The upper inset is the optical microscopy image of a graphene Hall bar FET on a SiO2/Si substrate. (b) Conductivity of graphene as a function of carrier density at room temperature. The black line of the experimental data is fitted by a Boltzmann model with red dots. (c) The density-dependent field-effect mobility of graphene plotted as a function of carrier density at room temperature. (d) Electrical properties of monolayer graphene Hall bar devices showing the half-integer quantum Hall effect, the longitudinal (Rxx) and transverse (Rxy) magnetoresistances are measured at 1.8 K under a magnetic fieldB=9 T. The half-integer plateaus corresponding tov=2, 6 and 10 are indicated by horizontal dash lines. Figure 3a displays a plot of resistivity of a graphene device, depending on the back gate voltage at room temperature. Figure 3b plots the conductivity as a function of carrier density n (defined by n=C g (V g −V D )/e , C g =11.5 nF cm −2 ), which shows that the conductivity ( σ ) is nearly linear with carrier density, with identical slopes for both electrons and holes. Figure 3c shows the carrier-density-dependent field-effect mobility ( μ FE =σ/ne ), ranging from ~11,000 cm 2 V −1 s −1 (at high carrier density 2 × 10 12 cm −2 ) to >14,000 cm 2 V −1 s −1 (at low carrier density 5 × 10 11 cm −2 ). We can also fit the conductivity data (red dashed line in Fig. 3b ) with a standard self-consistent diffusive transport model [28] , [29] , σ −1 =(neμ c +σ 0 ) −1 +ρ s , where μ c is defined as the carrier-density-independent carrier mobility corresponding to the long-range scattering, σ 0 is the residual conductivity at the Dirac point and the ρ s is the resistivity induced by the short-range scattering. The fitting gives a carrier-density-independent carrier mobility μ c =16,000 cm 2 V −1 s −1 , which is about 50% higher than the mobility reported in ref. 20 and comparable to those of the best exfoliated graphene samples on silicon oxide substrate [30] , [31] . This high carrier mobility achieved in our graphene devices demonstrates the excellent electronic quality of our graphene single crystals. In addition, the half-integer quantum Hall effect is clearly observed in the Hall bar device ( Fig. 3d ), further confirming that the electronic quality of the CVD graphene materials is comparable to that of the exfoliated graphene on the SiO 2 /Si substrate. Figure 3: Electronic properties. ( a ) Resistivity of graphene depending on the back-gate voltage at room temperature. The upper inset is the optical microscopy image of a graphene Hall bar FET on a SiO 2 /Si substrate. ( b ) Conductivity of graphene as a function of carrier density at room temperature. The black line of the experimental data is fitted by a Boltzmann model with red dots. ( c ) The density-dependent field-effect mobility of graphene plotted as a function of carrier density at room temperature. ( d ) Electrical properties of monolayer graphene Hall bar devices showing the half-integer quantum Hall effect, the longitudinal ( R xx ) and transverse ( R xy ) magnetoresistances are measured at 1.8 K under a magnetic field B =9 T. The half-integer plateaus corresponding to v =2, 6 and 10 are indicated by horizontal dash lines. Full size image It has been well recognized that the domain boundary is a primary factor responsible for the device-to-device variation in CVD graphene devices. The growth of giant graphene single crystals eliminates the domain boundaries and can greatly improve the device uniformity. To this end, we have fabricated a large number of graphene devices on a single crystalline domain. The electronic quality of a millimetre-sized monodomain was evaluated by measuring the back-gated field-effect transistors (FETs) produced on Si/SiO 2 substrates, using Ti/Au (50/50 nm) as the source and drain electrodes ( Supplementary Fig. S9 ). Two parallel samples of 55 transistors are fabricated on a 1-mm-sized single crystalline monodomain and a same-sized control sample of polycrystalline monolayer graphene sheet (with domain size of ~50 μm; the detailed growth processes are described in supporting information, see Supplementary Fig. S10 ). The transistor transport characteristics were studied in a probe station under ambient conditions to obtain the on-currents and carrier mobilities of all devices, which were used to create spatial distribution maps of the on-current and mobilities. Significantly, the devices fabricated from monodomain single crystal graphene sample show 100% yield with highly uniform distribution of the on-currents ( Fig. 4a ) and carrier mobilities ( Fig. 4d ) throughout the entire area. In contrast, the polycrystalline sample shows much larger variation in both the on-currents ( Fig. 4b ) and carrier mobilities ( Fig. 4e ). Overall, the mean values of on-currents and mobilities of the FETs from the single crystal sample are 173.8 μA and 6,391 cm 2 V −1 s −1 with s.d. of 22.3 μA and 843 cm 2 V −1 s −1 , respectively. In contrast, the mean values of the on-currents and mobilities of the FET arrays on polycrystalline sample are 98.7 μA and 3,601 cm 2 V −1 s −1 with s.d. of 51.4 μA and 1,941 cm 2 V −1 s −1 , respectively. It is noted that the carrier mobility values derived from these two terminal FET devices are generally lower than those of the four-terminal Hall bar devices, because the contribution of the contact resistance was not completely excluded here. Overall, the on-currents and mobilities of graphene FETs fabricated on small-domain-size polycrystalline samples show about 400% larger deviation (s.d. divided by mean value) than those on large-domain single crystalline graphene. This large deviation can be largely attributed to the domain boundary scattering, which does not exist in the large-domain graphene single crystals. 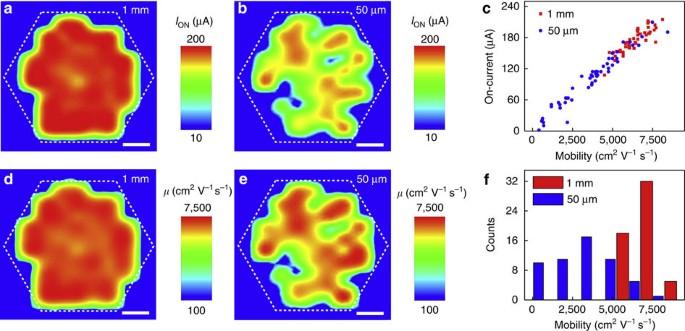Figure 4: Electronic uniformity of single crystalline versus polycrystalline graphene. (a) Two-dimensional colour plot of the on-current of a 55-FET-device array made on a 1-mm-sized single crystalline graphene monodomain and (b) on a 1-mm-area of polycrystalline graphene sheet (with individual domain size of ~50 μm). (c) On-currents and mobilities plot of the 55 FETs from the single crystalline graphene monodomain (red) and the polycrystalline graphene sheet (blue). (d) Two-dimensional colour plot of the hole mobility of the 55-FET-device array made on the single crystalline graphene monodomain and (e) on the same area polycrystalline graphene sheet. (f) Histogram of the carrier mobility distribution of the graphene FETs made on single crystalline domain (red) and polycrystalline sheet (blue). Scale bars, 200 μm ina,b,dande. Figure 4: Electronic uniformity of single crystalline versus polycrystalline graphene. ( a ) Two-dimensional colour plot of the on-current of a 55-FET-device array made on a 1-mm-sized single crystalline graphene monodomain and ( b ) on a 1-mm-area of polycrystalline graphene sheet (with individual domain size of ~50 μm). ( c ) On-currents and mobilities plot of the 55 FETs from the single crystalline graphene monodomain (red) and the polycrystalline graphene sheet (blue). ( d ) Two-dimensional colour plot of the hole mobility of the 55-FET-device array made on the single crystalline graphene monodomain and ( e ) on the same area polycrystalline graphene sheet. ( f ) Histogram of the carrier mobility distribution of the graphene FETs made on single crystalline domain (red) and polycrystalline sheet (blue). Scale bars, 200 μm in a , b , d and e . Full size image It is noted that the highest mobility value achieved in the polycrystalline sample (8,035 cm 2 V −1 s −1 ) is comparable to that in single crystalline sample (8,117 cm 2 V −1 s −1 ), whereas the lowest mobility observed in the polycrystalline sample (399 cm 2 V −1 s −1 ) is much lower than that in the single crystalline domain (4,495 cm 2 V −1 s −1 ). This is understandable, as the domain size of the polycrystalline sample (~50 μm) is larger than the device size (10 μm). In this case, for the polycrystalline samples a certain percentage of the devices are expected to have a single crystalline channel without domain boundaries to exhibit similar device characteristics to that of the large-domain single crystalline sample, whereas the other devices with domain boundaries in the channel exhibit much poorer device performance. It is also important to note that some extrinsic effects, such as the transfer process, surface-absorbed species or substrate–graphene interaction rather than the intrinsic quality of the graphene, could also contribute to the variation in mobility distribution or limit the highest mobility achievable in the devices without domain boundaries. To evaluate the overall quality of the continuous graphene film made of large-domain graphene, we have also compared the sheet resistances of the continuous graphene films formed by large domains (domain size of ~2 mm) and small domains (domain size of ~50 μm). To make more fair comparison between large-domain and small-domain devices, we took sheet resistance measurement on multidomain large-area sample (1 cm × 1 cm) so that the transport in both samples need to go across multiple domain boundaries. Here both large (~2 mm domain size) and small (~50 μm of lateral domain size) domain samples are polydomains, where large-domain sample has ~20–30 domains and small-domain sample has ~40,000 domains. Our studies clearly show that the overall sheet resistance of the large-domain sample is only about one quarter of that of the smaller domain samples ( Supplementary Fig. S11 ), which can be largely attributed to the greatly reduced domain boundary scattering in large-domain graphene film [32] . Growth of ultra-large bilayer graphene monodomains Using the very large single crystalline monolayer graphene domains as the templates, we can readily grow the second layer without crossing the boundary of the first layer, to achieve a large-domain bilayer graphene with consistent stacking order (for example, AB-stacking order, Supplementary Fig. S12a ) throughout the entire area. In contrast, for bilayer graphene obtained from small polydomain graphene, the stacking order can vary when the second layer goes across the grain boundary of the fist layer. To this end, we have carried out systematic time-dependent studies to investigate the growth kinetics of monolayer and bilayer graphene. In general, when the H 2 /CH 4 ratio is sufficiently high (for example, >6,600), the growth of bilayer graphene can be largely neglected. The growth of bilayer graphene became obvious with reducing H 2 /CH 4 ratio (for example, 4,400). Even under this condition, the growth of bilayer graphene is still about one order of magnitude slower than that of monolayer graphene ( Supplementary Fig. S12b ). This drastically different growth rate for the single and bilayer graphene can be attributed to a diffusion-limited growth. Specifically, all the active carbon species are generated by catalytically cracking CH 4 on the exposed Cu surface. For such carbon species to contribute to the growth of the second layer graphene, they have to diffuse across the edge of the first layer. In this process, most of such carbon species may be captured by the first layer and may contribute to the growth of the first layer. Only a small percentage of the carbon species may be able to go across the edge of the first layer to reach the second layer. The reduction of H 2 /CH 4 ratio can increase the supersaturation of the carbon precursors, to allow the active carbon species that have a greater chance to cross the edge of first layer and contribute to growth of the second-layer graphene ( Supplementary Fig. S12 ). On the other hand, it is also not practical to infinitely reduce the H 2 /CH 4 ratio and increase the supersaturation of the carbon precursors, which can lead to a rather fast growth of the first layer and a complete passivation of the entire Cu surface. The giant single crystals of monolayer graphene provide a perfect template for the growth of large-sized domains of bilayer graphene. For example, bilayer graphene domains can be readily obtained with the lateral size up to 300 μm without crossing any domain boundary on the first layer ( Supplementary Fig. S13 ). To the best of our knowledge, this is the largest AB-stacked bilayer domain ever reported to date [33] , [34] , [35] . A 200-μm bilayer graphene is evaluated by both the colour contrast under the optical microscope and more clearly the contrast shown in the SEM image ( Fig. 5a ). 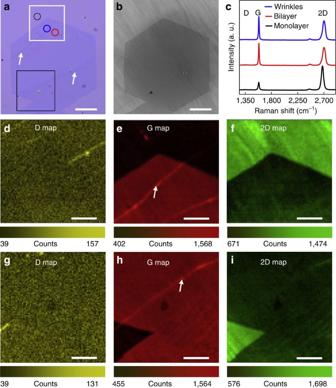Figure 5: Ultra-large monodomain of AB-stacked bilayer graphene. (a) Optical microscope image of a graphene domain transferred onto SiO2/Si substrate (300-nm-thick oxide layer) showing bilayer region (higher contrast hexagon at the centre of the image) and a few wrinkles formed during the transfer process (highlighted by white arrows). (b) SEM image of the same regions as ina. (c) Raman spectra taken from the marked spots with corresponding coloured circles ina; a.u., arbitrary units. (d–f) Raman maps of the D (~1,350 cm−1), G (~1,580 cm−1) and 2D (~2,680 cm−1) bands, respectively, obtained from the upper region of the bilayer graphene marked with white rectangle ina. (g–i) Raman maps of the D (~1,350 cm−1), G (~1,580 cm−1) and 2D (~2,680 cm−1) bands, respectively, obtained from the lower region of the bilayer graphene marked with black rectangles ina. The white arrows ineandhhighlight the wrinkles. Scale bars, 50 μm inaandb, 20 μm ind–i. Figure 5: Ultra-large monodomain of AB-stacked bilayer graphene. ( a ) Optical microscope image of a graphene domain transferred onto SiO 2 /Si substrate (300-nm-thick oxide layer) showing bilayer region (higher contrast hexagon at the centre of the image) and a few wrinkles formed during the transfer process (highlighted by white arrows). ( b ) SEM image of the same regions as in a . ( c ) Raman spectra taken from the marked spots with corresponding coloured circles in a ; a.u., arbitrary units. ( d – f ) Raman maps of the D (~1,350 cm −1 ), G (~1,580 cm −1 ) and 2D (~2,680 cm −1 ) bands, respectively, obtained from the upper region of the bilayer graphene marked with white rectangle in a . ( g – i ) Raman maps of the D (~1,350 cm −1 ), G (~1,580 cm −1 ) and 2D (~2,680 cm −1 ) bands, respectively, obtained from the lower region of the bilayer graphene marked with black rectangles in a . The white arrows in e and h highlight the wrinkles. Scale bars, 50 μm in a and b , 20 μm in d – i . Full size image Raman mapping experiment can be further used to identify the stacking order of the bilayer graphene. The Raman spectra of graphene show typical features of G (~1,580 cm −1 ) and 2D (~2,680 cm −1 ) bands. In general, the D bands (1,350 cm −1 ) are not visible for all samples, indicating the high quality of the resulting graphene with few defects. For single-layer graphene (black colour spectrum), the Raman spectrum shows 2D/G intensity ratio of 2.65 and the narrow symmetric 2D band (2,684 cm −1 ) with the full width at half-maximum of 33 cm −1 ( Fig. 5c ), consistent with the expected features of monolayer graphene. The darker hexagonal region in the centre of the optical image corresponds to the AB-stacked bilayer graphene ( Fig. 5a ). A typical spectrum (red colour spectrum) shows a wider and asymmetric 2D band (full width at half-maximum of 58 cm −1 ) with the 2D/G intensity ratio of about 0.8, which is quite similar to that of the exfoliated bilayer graphene samples with AB-stacking order [36] , [37] , [38] . Two sets of Raman maps were taken on both the upper (highlighted by white rectangles) and the lower region (highlighted by black rectangles) of the AB-stacked bilayer domain. The D map of the upper region of the domain is rather uniform and is at the background level ( Fig. 5d ), except for the area where wrinkles are present. No clear contrast is observed between the regions of monolayer and AB-stacked bilayer in D map, which indicates a similar good quality of the AB-stacked bilayer graphene to that of the monolayer. In the G map, the peak intensity of the AB-stacked bilayer graphene is about 2.2 times higher than that of monolayer region. In the 2D map, the peak intensity of the AB-stacked bilayer is about 71% compared with that of the monolayer region. These are clear signatures differentiating the AB-stacked bilayer from the monolayer graphene in the Raman maps. The wrinkles show a better contrast in the G map due to the large-intensity variations according to the number of the layers. The D, G and 2D maps of the lower region of the bilayer graphene domain are similar to that of the upper region ( Fig. 5g–i ). Within the two mapping regions (90 × 90 μm for each), the uniform of the peak heights observed in the monolayer and AB-stacked bilayer regions indicate high quality and good uniformity of our monolayer and bilayer graphene films. The Raman mapping confirms that a largest domain of AB-stacked bilayer graphene up to 300 μm can be achieved with our approach ( Supplementary Fig. S13 ). Electrical transport studies of the dual-gated AB-stacked bilayer graphene shows expected electrical characteristics, with the maximum Dirac resistance value increasing with V BG in both the positive and negative directions ( Supplementary Fig. S14 ). The emergence of quantum Hall effect at integer filling factors that are multiples of four, that is, ν =±4, ±8 ( Supplementary Fig. S14d ), is also consistent with the expected values in the exfoliated AB-stacked bilayer graphene, further confirming the AB-stacking order and the electronic quality of the bilayer graphene [39] , [40] . In summary, we have shown that the nucleation density of graphene domains in a CVD process can be dramatically reduced from ~10 6 to 4 nuclei cm −2 , using an integrated strategy of low reactor pressure, high hydrogen/methane molar ratio and pre-annealing of the copper foil in pure argon environment, and therefore enabling a straightforward way to prepare the largest single crystals of monolayer and bilayer graphene. The formation of ultra-large single crystalline graphene can enable excellent device performance with highly uniform electrical characteristics. It can therefore pave an effective pathway to large-scale integration of graphene devices with high yield and high reproducibility, which are the key to practical applications. Graphene growth Graphene was synthesized by copper-catalysed low-pressure CVD using a gas mixture of Ar, H 2 and diluted CH 4 (500 p.p.m. methane balanced in argon), where CH 4 gas was the carbon-containing precursor. First, 25-μm-thick copper foils (99.8%, Alfa Aesar, 13382) were washed by HCl/H 2 O (1:10), triple rinsed by isopropyl alcohol and dried by N 2 blow. The dried copper foils were loaded into a home-built CVD system in a horizontal tube furnace (Lindberg/Blue M) with 1-inch quartz tube. The system was pumped down to a vacuum of 10 mTorr in 30 min and refilled with 300 sccm of pure Ar gas or Ar/H 2 mixture and heated to 1,070 °C within 25 min (~20 min ramping time followed by ~5 min stabilization period). Next, the diluted methane and hydrogen was introduced into the CVD system for the graphene growth at 1,070 °C with different H 2 /CH 4 molar ratio (1,320~8,800) under variable pressure of 1–1,000 mbar. The growth was terminated by quenching the quartz tube (cooling rate was ~200 °C min −1 ) in ambient environment. Graphene transfer The transfer of the graphene films onto 300 nm SiO 2 substrates was performed by the wet-etching of the copper substrates. The graphene was grown on both sides of the copper foils, and one side of the graphene/copper surface was spin-coated with PMMA (poly(methyl methacrylate); 495 PMMA C2, MicroChem) and baked at 120 °C for 2 min. The other side of the sample was exposed to O 2 plasma for 60 s to remove the graphene. After that, the Cu foils were etched away using copper etchant (Transene, CE-100), resulting in a free-standing PMMA/graphene membrane floating on the surface of the etchant bath. The PMMA/graphene film was washed with HCl/deionized H 2 O (1:10) and deionized water for several times, and then transferred onto a silicon substrate with 300 nm SiO 2 . After air drying, the PMMA was dissolved by acetone and the substrate was rinsed with isopropyl alcohol to yield a graphene film on the substrate. Graphene device fabrication Single, back-gated and dual-gated graphene FETs were fabricated on the monolayer and bilayer graphene on a silicon substrate with 300 nm SiO 2 . To this end, the as-grown graphene is first transferred onto the blank Si/SiO 2 substrate. Photolithography and O 2 plasma etching were used to pattern graphene films into 7-μm-wide strips. After that, e-beam lithography was employed to pattern the contact electrodes with the channel lengths of 10 μm. The source/drain electrodes (Ti/Au: 50 nm/50 nm) were deposited using e-beam evaporation. The back-gate voltage was applied by using a Si back gate with SiO 2 as the dielectric. For the dual-gate device, a 30 nm Al 2 O 3 top dielectric layer was deposited on the top of device using e-beam evaporation, followed by the definition of top gate electrode (Ti/Au: 50 nm/50 nm) using e-beam lithography. Characterizations The morphology and structure of the graphene were characterized with optical microscopy (Olympus BX51 and Nikon), field emission SEM (JSM-6701F), high-resolution TEM (FEI Titan S/TEM at 300 kV) and Raman spectroscopy (Renishaw 1000, 514 nm laser wavelength, × 50 objective), Raman maps of the D (1,300−1,400 cm –1 ), G (1,560−1,620 cm –1 ) and 2D (2,660−2,700 cm –1 ) bands, respectively (514 nm laser wavelength, the Raman map pixel size is 1 μm). Electrical transport properties of the samples were measured at room temperature in a Lakeshore probe station (Model PTT4) with a computer-controlled analogue-to-digital converter (National Instruments model 6030E). How to cite this article: Zhou, H. et al. Chemical vapour deposition growth of large single crystals of monolayer and bilayer graphene. Nat. Commun. 4:2096 doi: 10.1038/ncomms3096 (2013).